The surface plasmon modes of self-assembled gold nanocrystals The three-dimensional (3D) self-assembly of nanocrystals constitutes one of the most important challenges in materials science. A key milestone is the synthesis of simple, regular structures, such as platonic solids, composed of nanocrystal building blocks. Such objects are predicted to have unique optical and electronic properties such as polarization-independent light-scattering and intense local fields. Here we present a two-stage process for fabricating well-defined and highly symmetric, 3D gold nanocrystal structures, including tetrahedra, 3D pentamers and 3D hexamers. Polarized scattering spectra are used to elucidate the plasmon modes present in each structure, and these are compared with computational models. We conclude that self-assembly of highly symmetric, polarization-independent structures with interparticle spacings of order 0.5 nm can now be fabricated. Drastically, enhanced local fields, 1000 times higher than the incident field strength, are produced within the interstices. Fano resonances are generated if the symmetry is broken. The crystallization of nanocrystals into two-dimensional (2D) [1] and three-dimensional (3D) [2] lattices has been studied for nearly 20 years. However, fabrication of arbitrary nanocrystal structures, such as cubes and prisms, composed of nanocrystal building blocks remains a fundamental scientific challenge. In the case of metal nanocrystals, one motivation for achieving such assembly is the possibility of creating materials with tunable optical resonances, which would facilitate the development of plasmonics. Surface plasmon resonances allow control of light below the diffraction limit and provide a potential platform for biosensing [3] , for fabrication of metamaterials [4] , [5] , [6] , [7] , [8] , nanocircuits [9] , subwavelength waveguides [10] , [11] , and nonlinear optics [12] . The coupling of surface plasmon modes is strongest at very small separations (<5 nm); however, it is extremely challenging to fabricate such systems by top-down lithography at present, even with high-resolution electron beam lithography. Conversely, colloidal particles spontaneously aggregate into dense, fractal-like structures [13] with very small separations (1–5 nm) that depend on the nature of the stabilizers present. Hence, colloidal assembly may provide an important fabrication method for plasmonic structures. In this paper, we utilize DNA-directed self-assembly to fabricate strongly coupled, 3D plasmonic structures for the first time. DNA-based assembly [14] has already generated considerable insight into one-dimensional [15] and 2D structures [16] , [17] , [18] , [19] , including the trimer, [18] tetramer [17] and pentamer [16] . 3D mesoscale tetrahedral and octahedral [20] systems have also been assembled using DNA as well as 2D [21] , [22] and 3D [23] , [24] lattices. However, although there have been reports of DNA-assembled 3D particle structures, they have invariably collapsed upon deposition onto a substrate, and no direct images of the structures could be obtained nor have optical studies been possible. [25] Hence, only electrostatically assembled 3D core-satellite superstructures have been fully characterized on a substrate, although these structures are highly asymmetric due to the random distribution of the satellite particles on the core. [26] We report here the first synthesis and optical studies of the plasmon modes of highly ordered 3D gold tetrahedra, pentamers and hexamers. The assembled structures are found to be stable on substrates in stark contrast to earlier clusters and can be visualized using scanning electron microscopy (SEM) and atomic force microscopy (AFM). Polarized and non-polarized spectra of individual structures are used to elucidate the plasmon modes present in each structure, which is then compared with computational (COMSOL) models. The fundamental question we aim to answer is whether chemical assembly can generate highly symmetric and polarization-independent superstructures. We utilize polarized light-scattering spectroscopy of single nanocrystal assemblies as a tool to monitor and analyse the processes of self-assembly and to prove that self-assembly can produce highly regular and uniform superstructures. DNA-mediated self-assembly method The two-stage assembly method used to make the 3D structures is outlined schematically in Fig. 1 . The first stage of the two-stage process is to form the base of the 3D nanostructures ( Fig. 1a ). Solutions of 30-nm gold nanoparticles, functionalized separately with S1, S3 and S4 oligonucleotides containing DNA base sequences designed to yield trimeric structures (the base ordering of each strand can be seen in Fig. 1e , along with a schematic of the complementarity of strands S1, S3 and S4 shown in Fig. 1f ) are mixed together. Following this, a phosphate-buffered saline (PBS) solution is added in order to initiate assembly, and the assembled structures are dip-coated onto 3-mercaptopropyltrimethoxysilane (MPS) functionalized indium tin oxide (ITO)-coated coverslips ( Fig. 1b ). We find that 5.6% of the resulting 2D assemblies are trimers and note that further purification techniques could be used to increase this yield, [27] although this was not carried out here. Following the formation of the base structures, the formed structures on the substrate were further functionalized with additional oligomer S1 ( Fig. 1c ) and then reacted with a solution of nanoparticles previously functionalized with the base-pair sequence complementary to S1 and S2 ( Fig. 1d ). Using this assembly method, the 3D structures are not assembled in solution, rather, they are built up step-wise on a substrate. 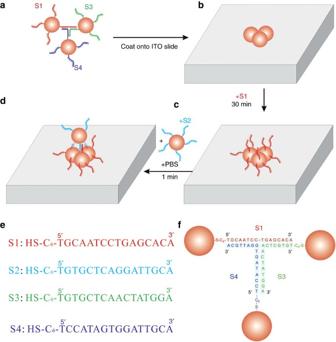Figure 1: DNA-meditated assembly scheme. (a) The hybridization mechanism is shown for producing the base of the 3D nanostructures. (b) Once assembled in solution, the bases of the 3D nanostructures are coated onto an ITO glass coverslip. (c) Structures that have been coated onto coverslips are then coated with a layer of thiolated DNA. (d) A second assembly step is then used to deposit a particle on top of the pre-coated structure. The base sequences of the DNA strands are shown in (e). (f) A schematic of the complementarity of strands S1, S3 and S4, which are used to make the base structures, is shown. Figure 1: DNA-meditated assembly scheme. ( a ) The hybridization mechanism is shown for producing the base of the 3D nanostructures. ( b ) Once assembled in solution, the bases of the 3D nanostructures are coated onto an ITO glass coverslip. ( c ) Structures that have been coated onto coverslips are then coated with a layer of thiolated DNA. ( d ) A second assembly step is then used to deposit a particle on top of the pre-coated structure. The base sequences of the DNA strands are shown in ( e ). ( f ) A schematic of the complementarity of strands S1, S3 and S4, which are used to make the base structures, is shown. Full size image SEM images of some 3D structures created using the self-assembly method depicted in Fig. 1 are shown in Fig. 2 , where each structure can be seen from above and from a 52-degree angle. As is evident in the SEM images, the tetramer consists of a 2D trimer base with a 4th particle resting on top and takes the form of a symmetric tetrahedron. In addition, 3D pentamer and hexamer structures are also formed. The pentamer consists of a 2D tetramer base with a 5th particle resting on top; and the hexamer consists of a 5 particle ring base with a 6th particle resting on top. In each case, the cap nanoparticle clearly rests in the interstices of the base structure. The yield of 3D tetramers is 1.0%, and that of 3D pentamers and hexamers are 1.1% and 0.15% respectively. Taking into account the initial yield of 2D trimers, the yield of 3D tetramers formed from these is 18%. 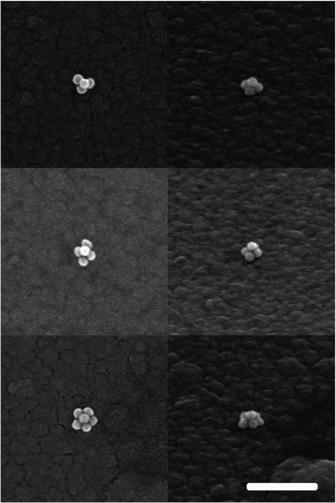Figure 2: SEM images of assembled nanostructures. A 3D tetramer (top), 3D pentamer (middle) and 3D hexamer (bottom) are shown. Each structure can be seen from both a top view (left column) and from a 52-degree angle (right column). Scale bar, 250 nm. Figure 2: SEM images of assembled nanostructures. A 3D tetramer (top), 3D pentamer (middle) and 3D hexamer (bottom) are shown. Each structure can be seen from both a top view (left column) and from a 52-degree angle (right column). Scale bar, 250 nm. Full size image The reason for 3D pentamer and hexamer formation is due to competing assembly pathways. The trimer forms only if single gold particles containing the S1, S3 and S4 strands assemble in solution. Statistically it is also possible for other base structures to form such as strings S1-S3-S1-S3. These will not form closed rings but form more open base structures. The string S1-S3-S1-S3-S4 will tend to form a closed pentamer. We show in Supplementary Fig. S1 of the Supplementary Information a number of different possible hybridization schemes that can lead to the formation of 2D tetramers and pentamers which form the base of the 3D pentamer and hexamer structures, although we note those shown are not exclusive. In addition to these structures, the formation of other lower-order (dimers) and higher-order aggregates occurs and lower-resolution SEM images of typical assembly results are shown in Supplementary Figs S2, S3, S4 and S5 . The use of the focussed ion beam correlation method [28] with single-particle spectroscopy allowed us to determine the scattering spectra of the 3D structures of interest. Comparing optical responses of 2D trimers and 3D tetramers We first consider the optical properties of a 2D equilateral trimer (shown in Fig. 3a ) under two typical polarization cases: p -polarization and s -polarization. In the s -polarization case ( k perpendicular to the substrate plane), the 2D equilateral trimer exhibits D 3 h symmetry and should display one in-plane electric dipolar bonding mode at lower energy than the triply degenerate single-particle plasmon mode [29] . This collective mode is predicted to possess a strong net dipole moment and will couple efficiently to the incident radiation. Consistent with this, we observe a strong scattering peak at about 705 nm as shown in Fig. 3c . The induced surface charge distributions are shown in the inset. These plots demonstrate that, in terms of the plasmon hybridization method, this mode belongs to the one of the degenerate E ′ eigenmodes [30] . Note that a magnetic mode ( A 2 ′ mode) with a ring-like arrangement of the dipoles is actually the lowest-energy eigenmode of this D 3 h cluster. However, it is unable to directly couple to the incident radiation (that is, it is a dark mode) and, hence, is not observed in the scattering spectrum. It is also pertinent to note that for the very small gaps present in these structures, quadrupole and octopole modes can also be excited, and we attribute the two minor peaks at about 585 and 548 nm to admixtures of such high-order modes, respectively (see Supplementary Fig. S6 ). 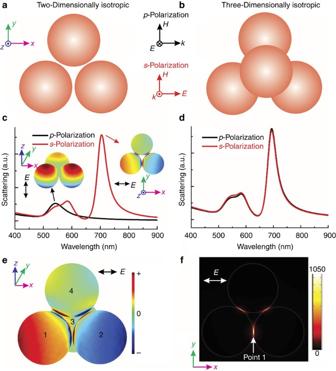Figure 3: Optical properties of a 2D trimer and a 3D tetramer. (a) A 2D equilateral trimer withD3hsymmetry and (b) A 3D symmetric tetramer. Two representative polarizations are indicated, which can induce out-of-plane and in-plane modes, respectively. (c) Theoretical scattering spectra for the 2D equilateral trimer underp- ands-polarizations. The insets show the surface charge distributions pictures at the relevant plasmon resonance wavelengths. (d) Scattering spectrum for 3D symmetric tetramer. (e) Calculated surface charge distributions diagram at the major scattering peak (λ=695 nm) unders-polarized incident light. (f) Map of the near-field electric field at the plane decided by the centres of the bottom trimer (sphere 1, 2 and 3) in the 3D tetramer when λ=695 nm. A significant hot spot is present at point 1. All particles in these models have a diameter of 30 nm and all interparticle spacings are 0.5 nm. Figure 3: Optical properties of a 2D trimer and a 3D tetramer. ( a ) A 2D equilateral trimer with D 3 h symmetry and ( b ) A 3D symmetric tetramer. Two representative polarizations are indicated, which can induce out-of-plane and in-plane modes, respectively. ( c ) Theoretical scattering spectra for the 2D equilateral trimer under p - and s -polarizations. The insets show the surface charge distributions pictures at the relevant plasmon resonance wavelengths. ( d ) Scattering spectrum for 3D symmetric tetramer. ( e ) Calculated surface charge distributions diagram at the major scattering peak (λ=695 nm) under s -polarized incident light. ( f ) Map of the near-field electric field at the plane decided by the centres of the bottom trimer (sphere 1, 2 and 3) in the 3D tetramer when λ=695 nm. A significant hot spot is present at point 1. All particles in these models have a diameter of 30 nm and all interparticle spacings are 0.5 nm. Full size image According to the plasmon hybridization method and group theory, light scattering from a completely symmetric trimer cluster should exhibit very little dependence upon the in-plane polarization angle of the excitation source. However, when the polarization is vertical to the substrate plane ( p -polarization with k parallel to the substrate plane), one out-of-plane bright mode appears at 545 nm as shown in the inset of Fig. 3c , which is blue-shifted with respect to the surface plasmon resonance of the single, uncoupled particle. The planar D 3 h cluster is only two-dimensionally isotropic. As shown in Fig. 3c , it still exhibits strong polarization-dependent scattering properties. Conversely, a 3D nanoparticle tetramer should exhibit completely 3D isotropic properties and is the smallest nanocrystal assembly, which does exhibit this property. Provided that the ensemble is much smaller than the wavelength of incident light, the optical response will be effectively isotropic and independent of the specific polarization and direction of the electromagnetic wave. As shown in Fig. 3d , the modelled scattering spectra from the 3D symmetric tetramer collected under light of two typical polarization cases nearly fully overlap, demonstrating that this 3D cluster is three-dimensionally isotropic. Until now, the only extant plasmonic structure that exhibited this fully isotropic characteristic was single-metal spheres. However, the 3D nanocrystal tetramer not only presents isotropic polarizability, perhaps more significantly, there will be a strong electric-field enhancement or hot spot produced in the interstices of the tetramer. As shown in Fig. 3f , the electric field at point 1 is calculated to be 1,000 times larger than the field of the incident light, although the use of the classical method at these small interparticle separations may overestimate the enhancement. [31] It is interesting to analyse the modes of the 3D symmetric tetramer. The surface charge distributions in spheres 4 and 3 (partly blocked) of Fig. 3e are exactly identical in the s -polarized case, which means that these two spheres have a similar role, whereas spheres 1 and 2 will largely determine the scattering intensity because of the strong dipole oscillations between them. These results are in accord with one of the T 2 modes obtained by the plasmon hybridization method. [6] Optical properties of the 3D tetramer The optical responses of an 3D tetramer and an SEM image of the structure are presented in Fig. 4a . The scattering spectra bands at around 550 nm at different polarization angles nearly fully overlap—these originate from coupling of several multipole modes, which makes peak positions difficult to measure. Although the resonance at about 700 nm exhibits a slight decrease in intensity, as well as a small blue shift of the peak position when the in-plane polarization angle changes from 0 to 90 degrees, we still believe this cluster must possess a high degree of morphological symmetry. In dark-field microscopy, even a slight change in focus may produce an observable intensity variation. In addition, the synthesized gold spheres are not completely spherical nor monodisperse, which must lead to some polarization anisotropy. From the simulations, there is no doubt that the optical properties of the nanoscale gold tetramer should be almost completely polarization angle independent, as shown in Fig. 4c . 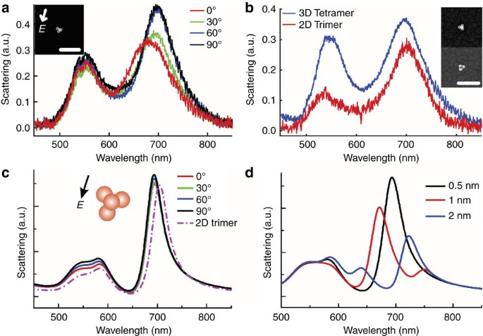Figure 4: Optical properties of the 3D tetramer. (a) Experimental scattering spectra for the 3D tetramer for different polarization directions (0, 30, 60 and 90 degrees). The inset shows an SEM image of the tetramer (Scale bar, 200 nm and the arrow indicates the polarization direction for 0 degrees). (b) Scattering spectra for 2D trimer and 3D tetramer. The insets show the relevant SEM images. All spectra were collected on ITO glass in immersion oil (refractive index=1.515) scale bar, 200 nm. (c) Calculated scattering spectra of a 3D symmetric tetramer at different polarization angles. The spectrum for a 2D equilateral trimer at 0 degree polarization is also included. (d) Calculated spectra of a 3D tetramer, where all spacings in the bottom trimer are fixed at 0.5 nm, and the gaps between the top sphere and bottom ones are varied from 0.5 nm (symmetric case) to 1 and 2 nm (symmetry breaking). Note that all the experimental spectra in this paper were measured unders-polarized incident light with an oblique angle of incidence (61 degrees), and the relevant modelling results are provided. Figure 4: Optical properties of the 3D tetramer. ( a ) Experimental scattering spectra for the 3D tetramer for different polarization directions (0, 30, 60 and 90 degrees). The inset shows an SEM image of the tetramer (Scale bar, 200 nm and the arrow indicates the polarization direction for 0 degrees). ( b ) Scattering spectra for 2D trimer and 3D tetramer. The insets show the relevant SEM images. All spectra were collected on ITO glass in immersion oil (refractive index=1.515) scale bar, 200 nm. ( c ) Calculated scattering spectra of a 3D symmetric tetramer at different polarization angles. The spectrum for a 2D equilateral trimer at 0 degree polarization is also included. ( d ) Calculated spectra of a 3D tetramer, where all spacings in the bottom trimer are fixed at 0.5 nm, and the gaps between the top sphere and bottom ones are varied from 0.5 nm (symmetric case) to 1 and 2 nm (symmetry breaking). Note that all the experimental spectra in this paper were measured under s -polarized incident light with an oblique angle of incidence (61 degrees), and the relevant modelling results are provided. Full size image As the gaps between the 3D tetramer are truly nanoscale, it is extremely difficult to experimentally determine the gap between the top particle and the bottom 2D trimer cluster. To verify that the tetramer is 3D symmetric, the relevant optical properties were modelled for various interparticle gaps (0.5, 1 and 2 nm). These calculations give a good indication of the sensitivity of the scattered spectrum to anisotropy in the structure. Breaking the D 3 h symmetry of such a cluster leads to strong coupling between the electric mode and the dark magnetic mode [32] . Accordingly, a Fano-like resonance dip appears at about 730 nm, which is simultaneously accompanied by two split scattering peaks, instead of the single scattering peak, resulting from coupled electric dipole modes in the fully symmetric 3D tetramer. The introduction of just a 0.5-nm gap change produces an enormous variation in the spectrum, which provides strong evidence that the tetramer is close to fully symmetric. When the spacing is further increased to 2 nm, an even more pronounced Fano resonance is observed, and the cluster spectrum totally differs from the symmetric case. We can conclude that the 3D tetramer shown here has high symmetry, with <0.5 nm deviation from ideal tetrahedral geometry. Figure 4b shows the experimental results for both the 3D tetramer and 2D trimer, which are in good agreement with the modelled results. One interesting point is that the major peak of the 3D tetramer shows a significant 10 nm blue-shift compared with the major peak of the 2D trimer. According to plasmon hybridization theory, the modes of complex nanostructures are equivalent to the electromagnetic interactions between plasmons of nanostructures of simpler geometry. Under the specific s -polarization case shown in Fig. 3b , the T 2 mode of the symmetric 3D tetramer can be approximated as a linear superposition of two identical trimers with E ′ mode symmetry. Thus, the origin of the blue shift is qualitatively similar to the case of a sphere dimer. Consequently, when the incident electric field is polarized perpendicularly to the major dimer axis, the scattering exhibits a small blue shift due to ‘dipole repulsion’, which is weakly dependent on the particle separation [27] , [33] . Optical properties of the 3D pentamer DNA self-assembly was also used to fabricate several other 3D structures. 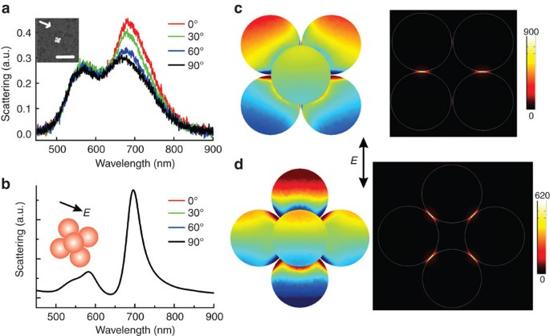Figure 5: Optical properties of the 3D pentamer. (a) Scattering spectra for a 3D pentamer versus polarization direction (0, 30, 60 and 90 degrees). Inset shows an SEM image of the tetramer (Scale bar, 200 nm and the arrow indicates 0 degrees polarization direction). All spectra were collected on ITO glass in immersion oil (refractive index=1.515). (b) Calculated scattering spectra for different polarization angles. All spectra overlap, highlighting the stability of the pentamers optical properties. Insets show the relevant 3D pentamer cluster, in which the bottom fours particles are arranged with square shape. (c,d) Surface charge distributions and electric field diagrams at the coupled electric dipolar resonance wavelength (695 nm), when polarization angle is 0 and 45 degrees, respectively. Figure 5a shows the optical responses of a 3D pentamer as a function of the polarization angle of the in-plane radiation. The spectra display a low-energy resonance at 678 nm and a high-energy resonance at 566 nm, which originate from the coupling of dipolar modes and high-order modes separately. In a similar fashion to the tetramer case, the peaks at 566 nm show little dependence on polarization, and the lower-energy peaks decrease in intensity and blue shift with changing polarization angle. Corresponding modelling, shown in Fig. 5b , clearly demonstrates that a symmetric pentamer should indeed exhibit no dependence on polarization angle for s -polarization (with the electric field oriented parallel to the substrate). It is worth pointing out that ordinarily two differently shaped structures can be formed when assembling 3D pentamers: in the first case, the four base particles form a square base (as shown in the inset of Fig. 5a ), and in the other case, the particles form a rhombic structure (see Supplementary Fig. S7 ). For the rhombic case, the upper particle cannot sit precisely in the centre of the bottom particles, and instead it will sit in one of the two vertices formed by three of the four base particles. Hence, the ‘rhombic pentamer’ should be inherently asymmetric. Accordingly, this cluster will exhibit pronounced polarization-sensitive effects, and this is borne out by the data shown in Supplementary Fig. S7 . Figure 5: Optical properties of the 3D pentamer. ( a ) Scattering spectra for a 3D pentamer versus polarization direction (0, 30, 60 and 90 degrees). Inset shows an SEM image of the tetramer (Scale bar, 200 nm and the arrow indicates 0 degrees polarization direction). All spectra were collected on ITO glass in immersion oil (refractive index=1.515). ( b ) Calculated scattering spectra for different polarization angles. All spectra overlap, highlighting the stability of the pentamers optical properties. Insets show the relevant 3D pentamer cluster, in which the bottom fours particles are arranged with square shape. ( c , d ) Surface charge distributions and electric field diagrams at the coupled electric dipolar resonance wavelength (695 nm), when polarization angle is 0 and 45 degrees, respectively. Full size image Figure 5c and d shows the calculated surface charge distributions and the magnitude of the electric field at 695 nm when the polarization angles are 0 and 45 degrees, respectively. Both the surface charge distributions exhibit electric dipolar modes that are strongly coupled (in phase), and these could be categorized as bonding modes. The electric-field-enhancement factors, relative to the field of the incident light, are obviously larger when the polarization angle is 0 rather than 45 degrees. Thus, in such a symmetric pentamer with s -polarization-independent scattering characteristics, the hot spots are polarization-selective. Optical properties of a 3D hexamer The DNA self-assembly method can also generate a 3D hexamer cluster. The experimentally determined scattering spectra of the hexamer as a function of polarization angle is shown in Fig. 6a . It is clear from this data that the spectra are relatively more polarization independent than both the tetramer and pentamer, which implies that the 3D hexamer is closer to fully symmetric. The theoretical scattering spectra in Fig. 6b are in good agreement with experiment. The obvious resonance at around 700 nm is due to coupling of the electric dipolar modes. 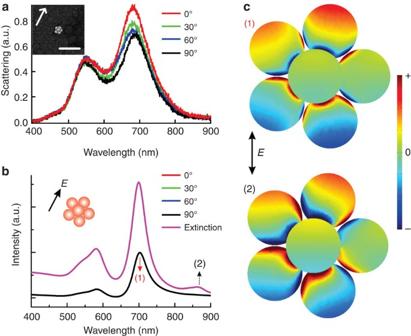Figure 6: Optical properties of a 3D hexamer. (a) Optical response of a 3D hexamer tos-polarized light. The inset shows an SEM image of the hexamer. Scale bar, 200 nm. Arrow direction indicates polarization direction for 0 degrees. All spectra were collected on ITO glass in immersion oil (refractive index=1.515). (b) Corresponding calculated results. All polarized spectra overlap, highlighting the optical stability of the structure. As the extinction spectra are in-plane polarization independent, only the extinction curve with polarization angle 0 degrees is shown. (c) Surface charge distributions at 705 nm (marked as (1)) and 870 nm (marked as (2)), respectively. Coupled charges oscillations oriented in the same direction and exhibit an enhanced electric mode in (1); surface charges oscillate circularly, which means a magnetic mode in (2). Figure 6c clearly depicts this enhanced electric ‘bright’ mode, where the surface charges are oriented in the same direction. The magnetic mode is supported by the outer ring of five nanospheres, which are arranged into a closed loop; therefore, it should effectively couple to the magnetic component of the incident electromagnetic field. However, similar to the magnetic dark modes for the circular 2D trimer, the magnetic mode has no net dipole moment, meaning it cannot couple to the incoming electromagnetic field and is therefore not visible in the scattering spectra. The simulated surface charge density of this mode is mapped out in Fig. 6c and shows circulating dipoles around the bottom 2D pentamer ring, which is characteristic of a magnetic dipole mode. The calculations indicate that the presence of the upper nanosphere does not affect the magnetic resonance of such a symmetric 3D hexamer cluster. This is quite different to the well-known planar symmetric heptamer, in which the middle nanoparticle has a great role and actually induces the occurrence of a Fano-like resonance by coupling the magnetic mode with the electric modes [34] . Figure 6: Optical properties of a 3D hexamer. ( a ) Optical response of a 3D hexamer to s -polarized light. The inset shows an SEM image of the hexamer. Scale bar, 200 nm. Arrow direction indicates polarization direction for 0 degrees. All spectra were collected on ITO glass in immersion oil (refractive index=1.515). ( b ) Corresponding calculated results. All polarized spectra overlap, highlighting the optical stability of the structure. As the extinction spectra are in-plane polarization independent, only the extinction curve with polarization angle 0 degrees is shown. ( c ) Surface charge distributions at 705 nm (marked as (1)) and 870 nm (marked as (2)), respectively. Coupled charges oscillations oriented in the same direction and exhibit an enhanced electric mode in (1); surface charges oscillate circularly, which means a magnetic mode in (2). Full size image However, it is again worth emphasizing that any symmetry breaking will also introduce strong coupling between these modes, and the corresponding spectra will then change dramatically. Note that the magnetic mode also exists in the 3D tetramer and pentamer cluster. These symmetric 3D magnetic molecules are two-dimensionally isotropic and, therefore, s -polarization-independent, which is extremely promising for constituting metamaterials with negative permeability [35] , negative refractive index [36] and other plasmonic applications. AFM measurements Finally, although the SEM can unambiguously show that 3D structures are formed, we have used tapping mode AFM to determine the actual morphology of individual structures. Typical images and cross-sections are presented in Supplementary Fig. S8 in the Supplementary Information . In Table 1 , we present the measured height of individual structures and compare them with the predictions for ideal geometries. Remarkably, given the 10% s.d. in the gold nanocrystal size distributions and the variations in spacing that occur with DNA assembly, the predicted and measured heights are within 5% for the tetramer, suggesting that the capping particles are firmly ensconced within the interstices, and this is entirely consistent with the polarization-independent properties found using dark-field spectroscopy. This suggests that following initial ‘contact hybridization’ of the gold particles, lateral diffusion over the base structure is possible to lower the free energy of the structure. The agreement is not as good for the pentamer and hexamer where the observed height is lower than predicted by geometry, indicating that there is some dilation of the base structures. Table 1 Tabulated results of AFM measurements. Full size table These results clearly demonstrate that DNA assembly can generate symmetric 3D nanocrystal superstructures with particle spacing in the 0.5–1 nm regime. We have presented one example of each structure, and it is pertinent to comment on the variations in the morphologies in the assemblies themselves. In Supplementary Figs S7, S9 and S10 , we present the optical properties of additional 3D structures (tetramer, pentamer and hexamer), along with SEM images of some other, less symmetric 3D assemblies in Supplementary Fig. S11 . The scattering spectra of the tetramer shown in Supplementary Fig. S9 exhibit a much larger polarization dependence than observed for the assembly in Fig. 4 . Our modelling predicts that the departure of even as little of 0.5 nm from ideal tetrahedral geometry leads to very large changes in the optical properties, including a large polarization dependence and the formation of a Fano-like resonance. For the tetramer shown in Supplementary Fig. S9 , a small dip in the middle of the lowest-energy resonance with polarization at 90 degrees is observed, consistent with the formation of a Fano-like resonance. The dependence of the scattering spectra on the polarization angle of the incoming s -polarization is also much larger than observed for the tetramer in Fig. 4 ; these features indicate that the assembly shown in Supplementary Fig. S9 has lower symmetry. It is notable that this greater asymmetry is not obvious from a comparison of the two SEM images. Conversely, the SEM images of the tetramer assemblies shown in Supplementary Fig. S11 do display a significantly greater degree of asymmetry. We therefore conclude that although highly symmetric tetramers are formed by DNA assembly, other, less symmetric structures are formed concomitantly. Dark-field spectra provide an ideal means by which to assess the symmetry of these structures. This is also the case for the pentamers, where a deviation from D 4 h symmetry in the base of the structure leads to two different possible vertices for the location of the top nanoparticle. In contrast, both the scattering spectra and the SEM images of the two hexamers ( Fig. 6 and Supplementary Fig. S10 ) indicate that they are more consistently symmetric than either of the other nanoassemblies and are therefore also more polarization angle independent. There are two factors that are crucial for the success of this assembly method. The first is that the base structures that are formed in the first assembly step should be geometrically close packed, with small interparticle spacings. Fortunately, these small spacings arise naturally due to the Van der Waals attraction between the gold particles and the repulsive interactions due to compression of the DNA strands. This balance determines the interparticle spacing. Clearly, the compressibility of the DNA layers will depend on the adsorption density of the strands, so uniform spacing requires uniform DNA densities on the particle surfaces. Perhaps, less obvious is that the gold particles in the second step will bind preferentially in the interstices of the base gold-particle structures. The fact that this seems to occur is attributed simply to the higher number of DNA strands that are accessible for binding when the particles adsorb symmetrically into the interstices. Thus, although it is also favourable for the capping particles to adsorb to the edges of the base structure, there is a significant fraction that do bind at the centre of the three-particle structure. We find that 5.6% of the 2D assemblies are trimers, which is not an unreasonable yield in a non-purified sample as each nanoparticle contains additional DNA strands that are also able to undergo hybridization with other nanoparticles containing complementary DNA. The trimer yield is able to be controlled somewhat by varying the hybridization time, and we find that a hybridization time of 1 min achieves good trimer yield while minimizing higher oligomer formation. Refining the assembly method [37] or utilizing previously established purification techniques [27] , [38] could be used to increase the yield of trimers and, subsequently, the yield of 3D tetramers. The yields obtained here for both the 2D trimers and 3D structures are relatively low; however, as noted, no attempt at structure purification was made. In the absence of the second DNA assembly step no 3D structures were observed to form (survey of 1,000 structures). In order to fully understand the optical properties of these 3D structures, we have theoretically studied the scattering spectra at different angles of incidence for two typical polarization cases ( s - and p -polarization), the tabulated results are shown in Supplementary Fig. S12 of the Supplementary Information . The results clearly show the 3D tetramer is three-dimensionally isotropic, whereas the 3D pentamer and hexamer are only two-dimensionally isotropic for s -polarized light, and the scattering will vary greatly when the angle of incidence changes for p -polarized light. Hence, the 3D tetramer, pentamer and hexamer exhibit 2D or 3D isotropic optical properties and hot spots. One potential application for the structures is the detection and spectroscopy of single molecules, in which the experimentally observed enhancement of Raman scattering with respect to an isolated molecule reaches 10 10 –10 11 (refs 39 , 40 ). Because the Raman enhancement is proportional to the fourth power of the local field, a local field with enhancement factor greater than approximately 500 should be created. This requirement cannot be met by a single sphere or other plasmonic structures fabricated by top-down approaches but is met by these 3D assemblies. We have demonstrated the first systematic synthesis of 3D, symmetric nanocrystal superstructures using DNA assembly, and demonstrated via single-particle spectroscopy that such strongly coupled structures can approach the degree of precision necessary for precise polarization control of incident light. Unlike previous work, the fabrication involves both solution phase conjugation and surface fabrication steps. Importantly, the ability to tune the spatial positioning with nanometre precision also enables materials with well-defined local-field enhancements to be created. Interestingly, classical electromagnetic models give excellent agreement with experiment, suggesting that even at 0.5–1 nm separations, 3D plasmon interactions remain in accord with classical electromagnetism theory. There is no need to invoke ‘tunnel plasmons’, which must form at even smaller separations than encountered here. The novel DNA-based assembly method developed here paves the way for fabricating other interesting plasmonic structures, such as chiral nanostructures. [41] , [42] Chemicals and gold nanosphere assembly Gold(III) chloride trihydrate (99.9+%) and tris(2-carboxyethyl)phosphine hydrochloride (TCEP) were purchased from Sigma Aldrich. All oligonucleotides were purchased from Geneworks. Cetyltrimethylammonium bromide was purchased from Ajax Chemicals. ITO coverslips were purchased from SPI. MPS was purchased from Sigma Aldrich. Spherical gold nanoparticles were prepared using the wet chemical synthesis developed by Rodriguez-Fernandez et al . [43] Briefly, citrate seeds were prepared by bringing 100 ml of aqueous 0.25 mM chloroauric acid (HAuCl4) to boiling temperature. Seed growth is initiated by the addition of 3.5 ml of aqueous 1 wt% sodium citrate solution. A deep red colour after 20 min of boiling indicates the presence of gold nanoparticle seeds. Growth solutions were then prepared by adding 1 ml of approximately 1 mM range concentration of aqueous HAuCl 4 to 88 ml of 0.015 M cetyltrimethylammonium bromide. A volume of 1 ml of ascorbic acid is then added. The concentration of ascorbic acid was adjusted so that a 2:1 ratio of ascorbic acid to HAuCl 4 was present. A volume of 10 ml of seed solution was then added to initiate growth of the seeds followed by stirring for a few minutes. The concentration of HAuCl 4 needed was calculated from the volume of gold required to grow the 17-nm diameter seeds to the desired diameter. Self-assembly The gold nanoparticles were assembled using thiol-terminated single-strand oligonucleotides via a two-stage assembly process, which is shown schematically in Fig. 1 . The first stage of the process was adapted from the work of Yao et al . [44] and is necessary to form the base of the 3D nanostructures. The same procedure was followed for all oligonucleotide strands to form nanoparticles functionalized with strands of the necessary oligonucleotide, which we label as S1, S3 and S4. To form the oligonucleotide functionalized nanoparticles, 5 μl of an oligonucleotide solution (100 μM in oligomer concentration, either S1, S2, S3 or S4) was added to 45 μl of a 200 μM TCEP solution. The resulting solution was left for 30 min to allow reduction of the terminal thiol moiety on the oligonucleotide. The reduced oligonucleotide solution was then added to 1000 μl of a solution of gold nanoparticles with 30 nm diameter and concentrations of approximately 6 × 10 10 particles per ml. Equal volumes of nanoparticles functionalized with S1, nanoparticles functionalized with S3 and nanoparticles functionalized with S4 were then mixed together, generally volumes of each sample between 250 and 500 μl were used. The trimer assembly reactions were initiated by adding 3 ml of 0.1 M PBS buffer to the mixed nanoparticles. After the assembly reaction had proceeded for 1 min, the assembled particles were dip-coated onto cleaned, MPS functionalized [45] ITO-coated glass coverslips to form the base of the 3D nanoparticle structures (see Fig. 1b ). Once the sample had been removed from the solution and dried under a stream of N 2 , it was placed in a water bath at room temperature and allowed to sit for 5 min, then removed and dried with a steady stream of N 2 . Once structures had been coated onto a coverslip to form the base of the 3D nanostructures, another 5 μl volume of oligonucleotide S1 was reduced in 45 μl of a 200 μM TCEP solution. After 30 min of reducing time, this solution was diluted to 1 ml and coated onto the coverslip by manual dropcasting. This solution was left on the coverslip for 30 min to allow the oligonucleotides to bind to the coated nanostructures, as seen in Fig. 1c . A volume of 1 ml of S2 functionalized gold nanoparticles (with complementary base pairing to oligonucleotide S1) was dropcast onto the previously formed base structures, and 6 ml of 0.1 M PBS solution was added to the solution on the slide to initiate the assembly ( Fig. 1d ). Once the reaction had proceeded for 30 s, the coverslip was removed from the reaction solution and dried with a gentle stream of N 2 . The sample was then placed in a water bath at room temperature and allowed to sit for 5 min, then removed and dried with a steady stream of N 2 . Characterization Individual 3D nanostructures were imaged using either an xT Nova Nanolab SEM or an FEI Helios 600 D545 and marked using a focused ion beam attachment to allow for pattern matching when viewing samples under a dark-field microscope [28] . Nanoparticle spectra were collected on a dark-field microscope (Nikon Ti-S). The white excitation light from a halogen lamp (25 W) was focussed onto the sample using a Nikon oil-immersion dark-field condenser. The scattered light was collected via a X100 Nikon CFI Plan Fluor oil-immersion objective with iris diaphragm (numerical aperture 0.5–1.3) and then focused onto the entrance slit of a MicroSpec 2150i imaging spectrometer coupled to a thermoelectrically cooled CCD (charge-coupled device) (Acton Pixis 1024B Exelon). Polarized scattering spectra were collected by rotating a polarizer (LPVIS 100, Thorlabs) into the light path just after the light source, which ensures that s -polarized incident light with an oblique incident angle of 61 degrees reaches the sample. All spectra were collected on ITO glass coverslips in immersion oil (refractive index=1.515). AFM measurements were carried out on a JPK Nano Wizard II AFM in tapping mode. The AC160TS cantilever (Veeco) used had a spring constant of ~42 N m −1 and a resonant frequency of 310 kHz. Modelling Finite-element method (COMSOL) was used to simulate the experimental results and to map the surface plasmon modes. In modelling, the particle clusters of interest were delimited by the perfectly matched layer (PML) method, which prevented any unwanted reflections through efficiently absorbing the scattering off the particles. All calculations were performed in an effective embedding medium n =1.515, to match experiment. The optical constants of gold were taken from Johnson and Christy [46] . S -polarized incident light with oblique incident angle 61 degrees to the normal of the substrate plane was chosen to strictly compare with the experiment results. Because the interparticle spacings could not be determined experimentally with sufficient precision, to fit the calculated spectra to experiment, we simulated clusters with different interparticle gaps, as shown in Supplementary Fig. S13 . Note that the tetramer with −2 nm spacing was also modelled, in which case the surface charge distributions at the major scattering peak wavelength are totally different to the non-touching case (as shown in Fig. 3e ). This control simulation strongly suggests there is no direct metal–metal contact in the nanocrystal assemblies. The gap is estimated to be 0.5 nm, which gives good agreement between calculation and experiment for all the 3D clusters (tetramer, pentamer and hexamer). How to cite this article: Barrow, S.J. et al . The surface plasmon modes of self-assembled gold nanocrystals. Nat. Commun. 3:1275 doi: 10.1038/ncomms2289 (2012).